NRBF2 regulates autophagy and prevents liver injury by modulating Atg14L-linked phosphatidylinositol-3 kinase III activity The Beclin 1-Vps34 complex, the core component of the class III phosphatidylinositol-3 kinase (PI3K-III), binds Atg14L or UVRAG to control different steps of autophagy. However, the mechanism underlying the control of PI3K-III activity remains elusive. Here we report the identification of NRBF2 as a component in the specific PI3K-III complex and a modulator of PI3K-III activity. Through its microtubule interaction and trafficking (MIT) domain, NRBF2 binds Atg14L directly and enhances Atg14L-linked Vps34 kinase activity and autophagy induction. NRBF2-deficient cells exhibit enhanced vulnerability to endoplasmic reticulum (ER) stress that is reversed by re-introducing exogenous NRBF2. NRBF2-deficient mice develop focal liver necrosis and ductular reaction, accompanied by impaired Atg14L-linked Vps34 activity and autophagy, although the mice show no increased mortality. Our data reveal a key role for NRBF2 in the assembly of the specific Atg14L-Beclin 1-Vps34-Vps15 complex for autophagy induction. Thus, NRBF2 modulates autophagy via regulation of PI3K-III and prevents ER stress-mediated cytotoxicity and liver injury. Autophagy is a conserved cellular pathway that degrades long-lived proteins and other cytoplasmic contents through lysosomes. Vps34 is the only class III phosphatidylinositol-3 kinase (PI3K-III) in mammals, it phosphorylates phosphatidylinositol to generate phosphatidylinositol-3 phosphate (PI(3)P) [1] . Beclin 1 is one of the earliest autophagy proteins identified in mammals [2] . The Beclin 1-Vps34 complex has an essential role in the autophagy nucleation and maturation process by forming multiple complexes with different binding partners. Previously, our group and others identified multiple Beclin 1-Vps34-binding partners, including Atg14L/Barkor [3] , [4] , [5] , UVRAG [6] , Rubicon [3] , [5] , Bif1 (ref. 7 ), AMBRA1 (ref. 8 ), Bcl2 (ref. 9 ) and others [10] . Despite the identification of an increasing number of Beclin 1-Vps34-interacting proteins, the molecular mechanism for their integral functions in regulating PI3K-III activity and autophagy remains poorly understood. UVRAG and Atg14L are known to directly bind Beclin 1 via their strong coiled-coil domain (CCD) interactions, forming stable Beclin 1-UVRAG and Beclin 1-Atg14L complexes, that are highly conserved and contribute to two distinct physiological functions of PI3K-III (ref. 11 ). The Atg14L complex controls initiation of autophagy [3] , [5] , whereas the UVRAG complex is involved predominantly in autophagosome maturation and endocytosis [12] . The Beclin 1-Vps34 complex is essential for mouse development and viability. The Beclin 1 or Vps34 knockout (KO) mice are early embryonic lethal [13] , [14] , [15] ; and liver-specific deletion of Vps34 leads to severe liver damage associated with hepatomegaly, hepatic steatosis and impaired protein degradation [16] . To elucidate the mechanism of PI3K-III-mediated autophagy regulation, we expanded our search for Beclin 1-Vps34 activity regulators and characterized their functions in vivo . Here we identify nuclear receptor binding factor 2 (NRBF2) as a Beclin 1-Vps34-binding protein [17] . NRBF2 modulates autophagy via regulating Atg14L-linked Vps34 activity. Our study also reveals a critical function of NRBF2 in promoting the assembly of a specific Atg14L-Beclin 1-Vps34-Vps15 complex as a highly active PI3K-III kinase complex. Our data demonstrate NRBF2 as a PI3K-III modulator that has a role in cell protection from ER stress-induced apoptosis and in tissue homeostasis. NRBF2 is a component of the Beclin 1-Vps34 complex Using green fluorescent protein-tagged Beclin 1 (Beclin 1-GFP) to replace the endogenous Beclin 1 in mice, we previously reported the identification of Atg14L, UVRAG, Rubicon and Vps15 proteins as Beclin 1-binding proteins (bands 1–6) ( Fig. 1a ) [5] . In the same experiment, we found a new Beclin 1-binding protein at 40 kDa (no. 7; Fig. 1a ), which was named NRBF2 in a previous publication and has little known function [17] . The interaction between endogenous Beclin 1 and NRBF2 was confirmed in mouse brain lysates through co-immunoprecipitation (IP) analysis with either anti-Beclin 1 or anti-NRBF2 antibody ( Fig. 1b ). Using anti-NRBF2 antibody IP, we found that NRBF2 is associated with Vps34, Vps15, Atg14L and UVRAG proteins in brain lysates, noting that all proteins, except UVRAG, are enriched after IP ( Fig. 1c ). In addition, gel filtration separating native protein complexes from mouse brain tissues according to protein size shows overlap of NRBF2, Atg14L and Beclin 1 proteins in multiple fractions. The ‘peak’ NRBF2 fractions correspond to a molecular weight of ~700 kDa ( Fig. 1d ), suggesting that the primary species of NRBF2 exist in large protein complexes. 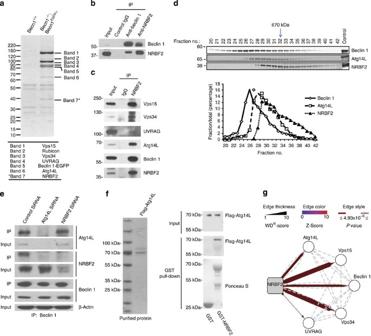Figure 1: Identification of NRBF2 as a novel component of Beclin 1-Vps34 complex. (a) Brains of the ‘rescued’ mice (Becn1−/−;Becn1EGFP/+) and of controlBecn1+/+littermates were lysed and subjected to immune isolation using an anti-GFP antibody. Proteins bound to anti-GFP antibody were isolated, detected and identified by SDS-PAGE, Coomassie brilliant blue staining and mass spectrometry. Seven bands pulled down by anti-GFP antibody specifically from ‘rescued’ mice lysate are numbered (this is a copy of image from our previous report with modification5). (b) Mouse brain lysates were subjected to co-immunoprecipitation (co-IP) followed by WB analysis using the indicated antibodies. (c) Mouse brain lysates were subjected to co-IP by NRBF2 antibody and followed by WB analysis using the indicated antibodies. (d) Gel filtration analysis. The supernatant fraction of mouse brain lysates was subjected to a Superdex 200 HR 10/30 column and each fraction was immunoblotted with the indicated antibodies. Relative amounts of each fraction determined by Odyssey software are plotted. (e) The deficiency of Atg14L impairs the protein interaction between Beclin 1 and NRBF2. NIH3T3 cells were transfected with Atg14L or NRBF2 RNAi for 72 h, respectively, and then were lysed and subjected to IP using Beclin 1 antibody. The immunoprecipitants were immunoblotted using the indicated antibodies. (f) Direct binding between Atg14L and NRBF2. Flag-tagged Atg14L purified from HEK293T cells overexpressing Flag-Atg14L was incubated with GST or NRBF2-GST purified fromEscherichia coli.The GST pull-down assay was performed to examine the direct binding between Flag-Atg14L and NRBF2-GST. (g) Proteomic analysis of NRBF2 interaction proteins. Association map shows identified high-confidence candidate interaction proteins (HCIPs). Liquid chromatography coupled to tandem mass spectrometry were performed to analyse the HA antibody-immunoprecipitated complexes derived from TREx-293 cells inducibly expressing HA-tagged NRBF2. Beclin 1, PIK3C3 (Vps34), PIK3R4 (Vps15) and Atg14L were detected as HCIPs in complex with NRBF2. Furthermore, UVRAG was detected with sub-threshold HCIP values. Dotted lines indicate interactions annotated in BIOGRID, MINT and HPRD protein interaction databases. The representative images shown in this figure are from two or three independent experiments. Figure 1: Identification of NRBF2 as a novel component of Beclin 1-Vps34 complex. ( a ) Brains of the ‘rescued’ mice ( Becn1 − / − ; Becn1 EGFP /+ ) and of control Becn1 +/+ littermates were lysed and subjected to immune isolation using an anti-GFP antibody. Proteins bound to anti-GFP antibody were isolated, detected and identified by SDS-PAGE, Coomassie brilliant blue staining and mass spectrometry. Seven bands pulled down by anti-GFP antibody specifically from ‘rescued’ mice lysate are numbered (this is a copy of image from our previous report with modification [5] ). ( b ) Mouse brain lysates were subjected to co-immunoprecipitation (co-IP) followed by WB analysis using the indicated antibodies. ( c ) Mouse brain lysates were subjected to co-IP by NRBF2 antibody and followed by WB analysis using the indicated antibodies. ( d ) Gel filtration analysis. The supernatant fraction of mouse brain lysates was subjected to a Superdex 200 HR 10/30 column and each fraction was immunoblotted with the indicated antibodies. Relative amounts of each fraction determined by Odyssey software are plotted. ( e ) The deficiency of Atg14L impairs the protein interaction between Beclin 1 and NRBF2. NIH3T3 cells were transfected with Atg14L or NRBF2 RNAi for 72 h, respectively, and then were lysed and subjected to IP using Beclin 1 antibody. The immunoprecipitants were immunoblotted using the indicated antibodies. ( f ) Direct binding between Atg14L and NRBF2. Flag-tagged Atg14L purified from HEK293T cells overexpressing Flag-Atg14L was incubated with GST or NRBF2-GST purified from Escherichia coli. The GST pull-down assay was performed to examine the direct binding between Flag-Atg14L and NRBF2-GST. ( g ) Proteomic analysis of NRBF2 interaction proteins. Association map shows identified high-confidence candidate interaction proteins (HCIPs). Liquid chromatography coupled to tandem mass spectrometry were performed to analyse the HA antibody-immunoprecipitated complexes derived from TREx-293 cells inducibly expressing HA-tagged NRBF2. Beclin 1, PIK3C3 (Vps34), PIK3R4 (Vps15) and Atg14L were detected as HCIPs in complex with NRBF2. Furthermore, UVRAG was detected with sub-threshold HCIP values. Dotted lines indicate interactions annotated in BIOGRID, MINT and HPRD protein interaction databases. The representative images shown in this figure are from two or three independent experiments. Full size image Atg14L binds NRBF2 directly and links NRBF2 to Beclin 1 We next examined the role of Atg14L in the NRBF2-Beclin 1 interaction. When Atg14L expression was knocked down with small interfering RNA (siRNA), anti-Beclin 1 antibody pulled down Beclin 1 but not NRBF2. The control scrambled siRNA treatment had no effect on the Beclin 1 and NRBF2 interaction ( Fig. 1e ). In contrast, NRBF2-specific siRNA treatment significantly reduced NRBF2 expression without altering the binding between Beclin 1 and Atg14L in the co-IP experiment ( Fig. 1e ). Thus, the Beclin 1-NRBF2 interaction critically depends on Atg14L. To characterize the Atg14L-NRBF2 interaction, we incubated purified FLAG-Atg14L protein with glutathione S-transferase (GST)-NRBF2 or control GST protein and performed a GST pull-down assay. GST-NRBF2, but not GST alone, pulled down FLAG-Atg14L, indicating a direct interaction between Atg14L and NRBF2 ( Fig. 1f ). We sought to identify sequence requirement(s) in Atg14L for the NRBF2-Atg14L binding. The results indicate that the N-terminal sequence of Atg14L that contains CCD 1 (1–95 amino acid) [5] is indispensable for the interaction between the two proteins ( Supplementary Fig. 1 ). Overexpressed NRBF2-CFP (cyan fluorescent protein) fusion protein was mostly diffused in the cytoplasm and nucleus in transfected HEK293 cells. When transfected alone, Beclin 1-GFP or Atg14L-AsRed also appeared to be diffused in the cytoplasm as previously shown [3] . But co-expression of NRBF2-GFP, Atg14L-AsRed and Beclin 1-Myc led to a redistribution of NRBF2-GFP into puncta also containing Atg14L-AsRed and Beclin 1-Myc ( Supplementary Fig. 2a,b ), suggesting an functional link between Atg14L, Beclin 1 and NRBF2 proteins. In a parallel experiment, we established a stable cell line expressing inducible hemagglutinin (HA)-tagged NRBF2 to identify NRBF2-binding proteins via HA affinity purification. The mass spectrometry analysis revealed Atg14L, Vps34, Vps15 and Beclin 1 proteins as the significant NRBF2-binding partners. Note that UVRAG was also found as an interactor of NRBF2, although with less confidence compared with the others ( Fig. 1g ), consistent with our findings from endogenous IP result ( Fig. 1c ). The above results identify NRBF2 as a new component in Beclin 1-Vps34 complexes associated primarily with Atg14L. NRBF2 MIT domain binds Atg14L to regulate Vps34 activity We then asked whether NRBF2 modulates PI3K-III activity. Because NRBF2 directly binds Atg14L ( Fig. 1 ), we specifically examined how loss of NRBF2 affects Atg14L-linked Vps34 activity. We first established mouse embryonic fibroblasts (MEFs) devoid of NRBF2 expression (KO) ( Supplementary Fig. 3 ). Using an anti-Atg14L antibody [18] , we performed IP to detect Atg14L-binding proteins in NRBF2 wild-type (WT) and KO MEFs. We found that levels of precipitated Vps34 and Vps15 are significantly reduced or diminished in NRBF2 KO cells when normalized against IPed Atg14L, while the total levels of these proteins are unchanged ( Fig. 2c ). We also analysed the precipitated Vps34 lipid kinase activity by measuring 32 P-labelled PI(3)P. The result showed that the Atg14L-linked Vps34 activity is markedly lower in NRBF2 KO MEFs than WT MEFs. Moreover, we re-introduced NRBF2 by transfecting NRBF2 KO MEFs with NRBF2-CFP and performed the same assays. We found that transfection of NRBF2-CFP, but not CFP, induces a recovery of Vps34 and Vps15 protein levels, as well as Vps34 lipid kinase activity in IP product of NRBF2 KO MEFs to near WT levels ( Fig. 2b,c ). 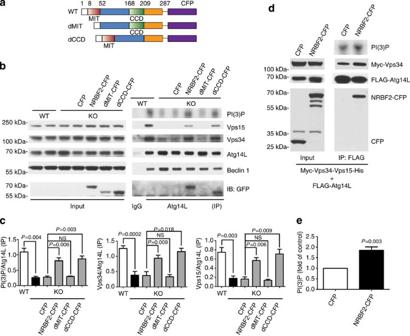Figure 2: NRBF2 modulates Atg14L-linked Vps34 lipid kinase activity through MIT domain. (a) The schematic map of full-length and truncate NRBF2-CFP. (b) NRBF2 KO MEFs were transfected with CFP, NRBF2-CFP, dMIT-CFP or dCCD-CFP for 48 h. Atg14L-linked Vps34 was pulled down by an anti-Atg14L antibody and subjected to KA. IP products and inputs were immunoblotted using the antibodies indicated. (c) Quantification of IPed Vps34 kinase activity (PI(3)P), Vps34 and Vps15 protein versus IPed Atg14L protein. (Data are shown as mean±s.e.m.,Pvalues are indicated on the figures, multiplet-test are followed by Bonferroni correction,n=4 (otherwise indicated,nmeans number of independent experiments; NS, not significant)). (b) Overexpression of NRBF2 enhances Atg14L-linked Vps34 kinase activity. HEK293T cells were co-transfected with Myc-Vps34-Vps15-His and Flag-Atg14L in the presence of CFP or NRBF2-CFP. Atg14L-linked Vps34 is pulled down by an anti-Flag antibody and subjected to KA (upper panel). IP products and inputs were immunoblotted using the antibodies indicated (upper panel). Quantification of Vps34 kinase activity (lower panel) shows the significant difference between two groups. (Data are shown as mean±s.e.m.,Pvalue is indicated on the figures, one samplet-test versus hypothetical mean 1,n=5). Figure 2: NRBF2 modulates Atg14L-linked Vps34 lipid kinase activity through MIT domain. ( a ) The schematic map of full-length and truncate NRBF2-CFP. ( b ) NRBF2 KO MEFs were transfected with CFP, NRBF2-CFP, dMIT-CFP or dCCD-CFP for 48 h. Atg14L-linked Vps34 was pulled down by an anti-Atg14L antibody and subjected to KA. IP products and inputs were immunoblotted using the antibodies indicated. ( c ) Quantification of IPed Vps34 kinase activity (PI(3)P), Vps34 and Vps15 protein versus IPed Atg14L protein. (Data are shown as mean±s.e.m., P values are indicated on the figures, multiple t -test are followed by Bonferroni correction, n =4 (otherwise indicated, n means number of independent experiments; NS, not significant)). ( b ) Overexpression of NRBF2 enhances Atg14L-linked Vps34 kinase activity. HEK293T cells were co-transfected with Myc-Vps34-Vps15-His and Flag-Atg14L in the presence of CFP or NRBF2-CFP. Atg14L-linked Vps34 is pulled down by an anti-Flag antibody and subjected to KA (upper panel). IP products and inputs were immunoblotted using the antibodies indicated (upper panel). Quantification of Vps34 kinase activity (lower panel) shows the significant difference between two groups. (Data are shown as mean±s.e.m., P value is indicated on the figures, one sample t -test versus hypothetical mean 1, n =5). Full size image There are two discrete motifs in NRBF2: an N-terminal MIT domain and a C-terminal CCD ( Fig. 2a ). We transfected NRBF2 KO MEFs with NRBF2 mutants missing either the MIT domain (dMIT-CFP) or the CCD (dCCD-CFP), and performed IP and lipid kinase assays (KAs) as described above. The result shows that both full-length NRBF2-CFP and dCCD-CFP mutant were pulled down together with endogenous Atg14L by anti-Atg14L antibody, which is associated with the enhanced Vps34 and Vps15 protein levels and lipid kinase activity. In contrast, the dMIT-CFP mutant fails to interact with Atg14L or rescue Vps34/Vps15 levels in NRBF2 KO MEFs ( Fig. 2b ). The data demonstrate that Atg14L interacts with NRBF2 through its MIT domain and promotes Vps34-Beclin 1-Vps15-Atg14L complex formation required for modulating Atg14L-linked Vps34 activity. To further assess NRBF2’s role in modulating Atg14L-Vps34 activity, we overexpressed NRBF2-CFP together with Myc-Vps34, Vps15-V5-His and FLAG-Atg14L in HEK293T cells and measured FLAG-Atg14L-linked Vps34 kinase activity. The result shows that NRBF2-CFP expression increases the 32 P-PI(3)P levels above the control CFP transfection ( Fig. 2d,e ). The data strongly support the role of NRBF2 in promoting Atg14L-linked Vps34 activity. NRBF2 regulates autophagy induction We observed NRBF2-GFP co-localization with Atg14L-AsRed and Beclin1-Myc in puncta to which autophagosome protein LC3 appears to be recruited in both normal and nutrient starvation conditions ( Supplementary Fig. 2c ). To determine the role of NRBF2 in autophagy, we first examined the impact of NRBF2 knockdown on long-lived protein degradation. When grown in complete medium, NIH3T3 cells treated with NRBF2 siRNA displayed a trend of reduction in the 3 H-leucine release compared with the cells treated with control siRNA. Upon nutrient starvation, NRBF2 siRNA caused a significant decrease in 3 H-leucine release, while this effect was abolished in the presence of wortmannin, an inhibitor of PI3K-III and autophagy ( Fig. 3a ). Atg14L knockdown with siRNA showed a similar effect to NRBF2 siRNA in impairing autophagic activity as expected ( Fig. 3a ). 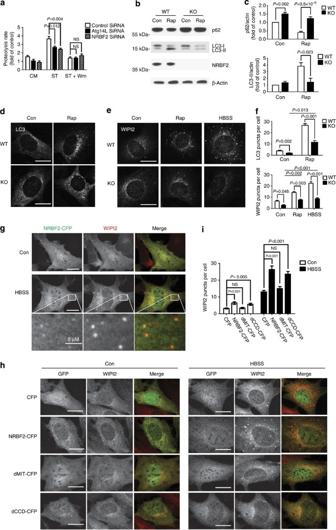Figure 3: NRBF2 regulates autophagy induction. (a) Starvation-induced long-lived protein degradation is impaired after NRBF2 knockdown. Compared with control (con) siRNA, NRBF2 siRNA decreases long-lived protein degradation (proteolysis rate) in NIH3T3 cells under starvation (ST) condition. This difference is diminished when the starved cells are co-treated with wortmannin (WM, 100 nM). (Data are shown as mean±s.e.m.,Pvalues are indicated on the figures, one-way analysis of variance with Dunnett aspost hoctest,n=4; NS, not significant). (b) Rapamycin (Rap)-induced autophagy is impaired in the NRBF2 KO cells. The MEFs were treated with (dimethyl sulfoxide) DMSO or 50 μg ml−1of Rap for 4 h then the cell lysates were immunoprobed with anti-LC3 and anti-p62 antibodies. (c) LC3-II and p62 levels were quantified and normalized with β-actin. Quantification results show that Rap-induced LC3 lipidation (upper) and p62 degradation (lower) were markedly impaired in the NRBF2 KO MEFs. (Data are shown as mean±s.e.m.,Pvalues are indicated on the figures, one samplet-test (WT con versus KO con) or unpairedt-test (WT Rap versus KO Rap)). p62 blots quantification,n=6; LC3 blots quantification,n=3). (d,e) The MEFs were subjected to Rap (50 μg ml−1) or starvation (HBSS) treatment then stained with anti-LC3 (d) or anti-WIPI2 (e) antibody. (f) The LC3 and WIPI2 puncta per cell were counted and quantified. (Data are shown as mean±s.e.m.,Pvalues are indicated on the figures, independent samples Kruskal–Wallis test followed by pairwise comparisons,n=30 randomly selected cells, a representative result from three independent repeats). (g) NRBF2-CFP stable cells were starved in HBSS for 4 h and then subjected to WIPI2 staining. Under starved condition, NRBF2-CFP forms puncta structures that co-localized with WIPI2. This is a representative image from three independent experiments. (h) The NRBF2 KO MEFs were transfected with CFP, NRBF2-CFP, dMIT-CFP or dCCD-CFP for 24 h and then followed by co-immunostaining with GFP and WIPI2 antibodies. (i) The WIPI2 puncta number per cell in GFP-positive cells were counted and quantified. (Data are shown as mean±s.e.m.,Pvalues are indicated on the figures, independent samples Kruskal–Wallis test followed by pairwise comparisons,n=30 randomly selected cells, a representative result from two independent repeats). Scale bars, 20 μm, or length indicated on the figure. CM, culture medium. Figure 3: NRBF2 regulates autophagy induction. ( a ) Starvation-induced long-lived protein degradation is impaired after NRBF2 knockdown. Compared with control (con) siRNA, NRBF2 siRNA decreases long-lived protein degradation (proteolysis rate) in NIH3T3 cells under starvation (ST) condition. This difference is diminished when the starved cells are co-treated with wortmannin (WM, 100 nM). (Data are shown as mean±s.e.m., P values are indicated on the figures, one-way analysis of variance with Dunnett as post hoc test, n =4; NS, not significant). ( b ) Rapamycin (Rap)-induced autophagy is impaired in the NRBF2 KO cells. The MEFs were treated with (dimethyl sulfoxide) DMSO or 50 μg ml −1 of Rap for 4 h then the cell lysates were immunoprobed with anti-LC3 and anti-p62 antibodies. ( c ) LC3-II and p62 levels were quantified and normalized with β-actin. Quantification results show that Rap-induced LC3 lipidation (upper) and p62 degradation (lower) were markedly impaired in the NRBF2 KO MEFs. (Data are shown as mean±s.e.m., P values are indicated on the figures, one sample t -test (WT con versus KO con) or unpaired t -test (WT Rap versus KO Rap)). p62 blots quantification, n =6; LC3 blots quantification, n =3). ( d , e ) The MEFs were subjected to Rap (50 μg ml −1 ) or starvation (HBSS) treatment then stained with anti-LC3 ( d ) or anti-WIPI2 ( e ) antibody. ( f ) The LC3 and WIPI2 puncta per cell were counted and quantified. (Data are shown as mean±s.e.m., P values are indicated on the figures, independent samples Kruskal–Wallis test followed by pairwise comparisons, n =30 randomly selected cells, a representative result from three independent repeats). ( g ) NRBF2-CFP stable cells were starved in HBSS for 4 h and then subjected to WIPI2 staining. Under starved condition, NRBF2-CFP forms puncta structures that co-localized with WIPI2. This is a representative image from three independent experiments. ( h ) The NRBF2 KO MEFs were transfected with CFP, NRBF2-CFP, dMIT-CFP or dCCD-CFP for 24 h and then followed by co-immunostaining with GFP and WIPI2 antibodies. ( i ) The WIPI2 puncta number per cell in GFP-positive cells were counted and quantified. (Data are shown as mean±s.e.m., P values are indicated on the figures, independent samples Kruskal–Wallis test followed by pairwise comparisons, n =30 randomly selected cells, a representative result from two independent repeats). Scale bars, 20 μm, or length indicated on the figure. CM, culture medium. Full size image Under both normal (full medium) conditions and rapamycin treatment (a stimulator of autophagy), NRBF2 KO MEFs have higher levels of autophagy substrate p62/SQSTM1 than WT MEFs ( Fig. 3b,c ). Although the levels of the lipidated form of LC3 (LC3-II) are similar between NRBF2 KO and WT MEFs under normal conditions, rapamycin treatment results in a significant increase in LC3-II levels in WT MEFs but not in NRBF2 KO MEFs. Furthermore, induced expression of AcGFP-NRBF2 in a stably transfected cell line leads to an increase in both LC3-I and LC3-II levels ( Supplementary Fig. 3 ). We next examined phagophores (autophagosome precursors) and autophagosome numbers in NRBF2 KO MEFs. The number of autophagosomes labelled by anti-LC3 antibody was decreased in NRBF2 KO MEFs compared with WT MEFs under normal conditions and rapamycin treatment ( Fig. 3d,f ). Staining phagophores with anti-WIPI2 antibody shows remarkable reduction of fluorescent puncta under normal condition, rapamycin treatment and nutrient withdrawal (Hank's Balanced Salt Solution (HBSS) buffer) in NRBF2 KO MEFs compared with WT MEFs ( Fig. 3e,f ). Induction of autophagy with rapamycin or HBSS buffer increased LC3 and WIPI2 puncta in NRBF2 KO MEFs but to a much lesser extent than WT MEFs. In addition, the difference in WIPI2 puncta number between KO and WT MEF is much more robust with rapamycin treatment or HBSS than under control or non-stressful condition (one-way analysis of variance; P =0.003 and P =0.001 versus P =0.045). We thus conclude that NRBF2 positively regulates autophagic activity and is particularly important for induced autophagy. WIPI2 structure formation depends on NRBF2 We established a ‘revertant’ stable cell line expressing NRBF-CFP in NRBF2 KO background to examine the subcellular localization of NRBF2-CFP. Under normal conditions, NRBF2-CFP distribution is diffuse. Upon autophagy induction (HBSS buffer), NRBF2-CFP redistributes to puncta that are positive for WIPI2 ( Fig. 3g ). Consistently, transient transfection of NRBF2-CFP in NRBF2 KO cells results in co-localization of NRBF2-CFP and WIPI2 in puncta that are also labelled with p62 upon autophagy induction ( Supplementary Fig. 2d ). Since deletion of NRBF2 decreases WIPI2-associated phagophore formation, we ask whether reintroduction of NRBF2 can rescue the defect. We transfected NRBF2 KO cells with NRBF2-CFP, NRBF2-CFP mutants or CFP, and quantified WIPI2 puncta. NRBF2-CFP and dCCD-CFP mutant transfections cause a significant increase in the number of WIPI2 puncta compared with CFP transfection under both normal and HBSS conditions. In contrast, dMIT-CFP transfectants have similar numbers of WIPI2 puncta to the CFP-transfected NRBF2 KO MEFs ( Fig. 3h,i ). The data suggest that expression of full-length NRBF2 or dCCD mutant rescues impaired WIPI2 formation in NRBF2 KO MEFs. Thus, the MIT domain of NRBF2, but not the CCD, is critical for the formation of WIPI2-associated phagophores after autophagy induction. Role of NRBF2 in modulating UVRAG-linked Vps34 activity We examined the role of NRBF2 in autophagosome maturation by using the tandem reporter mCherry-GFP-LC3B [19] . The dual colour fluorescent LC3 becomes red when labelling mature autophagosomes because of the acidic environment, whereas it remains in yellow (presence of both green and red colour) when localized in immature autophagosomes [19] , [20] . Our results show that the number of red LC3 puncta per cell and red LC3 puncta percentage are both reduced in NRBF2 KO MEFs under normal conditions. The differences in red-only LC3 puncta and red-only LC3 percentage between NRBF2 KO and WT MEFs are much more robust with rapamycin treatment (or nutrient starvation) compared with that under normal medium ( Fig. 4a,b ). This finding demonstrates impaired autophagosome maturation in the absence of NRBF2, particularly under autophagy induction. Moreover, we found that red fluorescent protein tagged LC3 (RFP-LC3) puncta rarely recruited the lysosomal marker LAMP2 in NRBF2 KO MEFs expressing RFP-LC3, whereas RFP-LC3-labelled autophagosomes have extensive overlap with LAMP2 in WT MEFs ( Fig. 4c ). 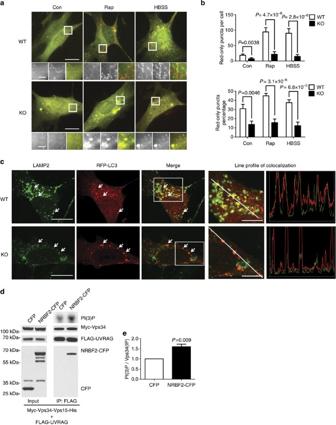Figure 4: NRBF2 is involved in autophagosome maturation. (a) NRBF2 KO MEFs display impaired autophagosome acidification. WT and NRBF2 KO MEFs are transiently transfected with mCherry–GFP–LC3B. WT MEFs expressing mCherry–GFP–LC3B contain many red-only puncta along with yellow (presence of both red and green) puncta. The number of both red-only puncta and yellow puncta markedly increases after rapamycin (Rap; 50 μg ml−1, 4 h) or starvation (HBSS, 4 h) treatment, suggesting the increased autophagolysosomes and nascent autophagosomes. In contrast, NRBF2 KO MEFs expressing mCherry–GFP–LC3B contain quite fewer red-only puncta and yellow puncta, even after Rap or starvation treatment. (b) The quantification results show that both the numbers of red-only puncta and percentage of red-only puncta (verses total puncta) in KO MEFs were markedly reduced. (Data are shown as mean±s.e.m.,Pvalues are indicated on the figures, Mann–WhitneyU-test,n=20 randomly selected cells, a representative result from three independent repeats), indicating both the autophagolysome number and autophagosome acidification rate are reduced in KO cells. Scale bars, 20 μm or 10 μm (amplified regions). (c) Autophagolysome formation is impaired in NRBF2 KO MEFs. WT and NRBF2 KO MEFs were transiently transfected with RFP-LC3 then stained with LAMP2 antibody. The co-localization between RFP-LC3 and LAMP2 are illustrated by line profile. RFP-LC3 puncta recruit much stronger LAMP2 signal in WT MEFs than in NRBF2 KO MEFs (as indicated by white arrows), suggesting the impairment of autophagolysosome formation in KO cells. Scale bars, 20 μm or 10 μm (amplified regions). This is a representative image from three independent experiments. (d) Overexpression of NRBF2 enhances UVRAG-linked Vps34 kinase activity. HEK293T cells were co-transfected with Myc-Vps34-Vps15-His and FLAG-UVRAG, in the presence of CFP or NRBF2-CFP. UVRAG-linked Vps34 was pulled down by an anti-FLAG antibody and subjected to KA. IP products and inputs are immunoblotted using the antibodies indicated. (e) Quantification of Vps34 kinase activity normalized with immunoprecipitated Vps34 shows the significant difference between two groups. (Data are shown as mean±s.e.m.,Pvalue is indicated on the figures, one samplet-test versus hypothetical mean 1,n=5). Figure 4: NRBF2 is involved in autophagosome maturation. ( a ) NRBF2 KO MEFs display impaired autophagosome acidification. WT and NRBF2 KO MEFs are transiently transfected with mCherry–GFP–LC3B. WT MEFs expressing mCherry–GFP–LC3B contain many red-only puncta along with yellow (presence of both red and green) puncta. The number of both red-only puncta and yellow puncta markedly increases after rapamycin (Rap; 50 μg ml −1 , 4 h) or starvation (HBSS, 4 h) treatment, suggesting the increased autophagolysosomes and nascent autophagosomes. In contrast, NRBF2 KO MEFs expressing mCherry–GFP–LC3B contain quite fewer red-only puncta and yellow puncta, even after Rap or starvation treatment. ( b ) The quantification results show that both the numbers of red-only puncta and percentage of red-only puncta (verses total puncta) in KO MEFs were markedly reduced. (Data are shown as mean±s.e.m., P values are indicated on the figures, Mann–Whitney U -test, n =20 randomly selected cells, a representative result from three independent repeats), indicating both the autophagolysome number and autophagosome acidification rate are reduced in KO cells. Scale bars, 20 μm or 10 μm (amplified regions). ( c ) Autophagolysome formation is impaired in NRBF2 KO MEFs. WT and NRBF2 KO MEFs were transiently transfected with RFP-LC3 then stained with LAMP2 antibody. The co-localization between RFP-LC3 and LAMP2 are illustrated by line profile. RFP-LC3 puncta recruit much stronger LAMP2 signal in WT MEFs than in NRBF2 KO MEFs (as indicated by white arrows), suggesting the impairment of autophagolysosome formation in KO cells. Scale bars, 20 μm or 10 μm (amplified regions). This is a representative image from three independent experiments. ( d ) Overexpression of NRBF2 enhances UVRAG-linked Vps34 kinase activity. HEK293T cells were co-transfected with Myc-Vps34-Vps15-His and FLAG-UVRAG, in the presence of CFP or NRBF2-CFP. UVRAG-linked Vps34 was pulled down by an anti-FLAG antibody and subjected to KA. IP products and inputs are immunoblotted using the antibodies indicated. ( e ) Quantification of Vps34 kinase activity normalized with immunoprecipitated Vps34 shows the significant difference between two groups. (Data are shown as mean±s.e.m., P value is indicated on the figures, one sample t -test versus hypothetical mean 1, n =5). Full size image Because the reduced Atg14L-linked Vps34 activity may not explain the impaired autophagy maturation in NRBF2 KO cells, we then asked whether NRBF2 regulates UVRAG-associated Vps34 activity, which is known to regulate autophagosome maturation. In fact, our study revealed a weak interaction between NRBF2 and UVRAG ( Fig. 1c,g ). We evaluated UVRAG-linked Vps34 activity like we did for Atg14L by transfecting Myc-Vps34/Vps15-His, FLAG-UVRAG and NRBF2-CFP or CFP, followed by IP with anti-FLAG antibody and measuring precipitated Vps34 activity. The result showed that the FLAG-UVRAG-linked Vps34 activity is significantly higher in the presence of overexpressed NRBF2-CFP than control CFP ( P value=0.009) ( Fig. 4e ). The data suggest that NRBF2 positively regulates UVRAG-linked Vps34 activity, providing a possible explanation for the impaired autophagosome maturation without NRBF2. NRBF2 KO mice develop focal liver necrosis We generated NRBF2 KO mice that do not express NRBF2 protein in multiple tissues ( Supplementary Fig. 4 ). In contrast to Beclin 1 KO [13] or Atg14L KO mice, which are both lethal at early embryonic development (our unpublished data), NRBF2 KO mice are born normally with a typical Mendelian ratio (data not shown). Surprisingly, the NRBF2 null mutant mice did not display overt abnormalities based on appearance and they show no enhanced mortality compared with their WT littermates and survived for up to 12 months ( n >20; Supplementary Fig. 5a,b ). We first focused our study on the livers of NRBF2 KO mice. The general appearance, size and liver index (ratio of liver mass to body mass) of the KO mice are similar to those of WT at 10 months ( Fig. 5a ). Histological examination with haematoxylin and eosin staining showed grossly normal lobules structures and hepatocytes in KO liver. However, we found isolated hepatocyte necrosis (red arrow) and focal ductular reaction (non-specific liver injury marker; yellow arrow) ( Fig. 5b ) in KO liver. The necrosis was confirmed by lymphocyte marker CD45 staining (black arrow); these abnormal structures were much more frequent in KO than WT livers ( Fig. 5c ). This data thus suggest that deletion of NRBF2 caused liver necrosis, albeit limited and without mortality up to 12 months. 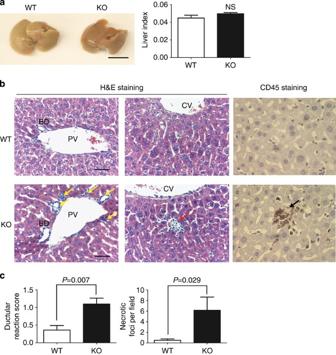Figure 5: NRBF2 KO mice have no enhanced mortality but with focal liver nercrosis. (a) The gross anatomical views of representative 4% paraformaldehyde-fixed livers and quantification of liver index. (Data are shown as mean±s.e.m.,Pvalues are indicated on the figures, unpaired Student’st-test,n=3 mice each group). Scale bar, 1 cm. (b) The haematoxylin and eosin (H&E) and CD45 staining of 10-month-old WT and NRBF2 KO mice livers. The NRBF2 KO liver shows mild increase of ductular reaction (yellow arrow) and isolated necrosis (red arrows). The necrotic foci were further confirmed by CD45 staining (black arrow). This is a representative image from four mice per genotype. Scale bar, 50 μm. (c) The number of necrotic foci and ductular reaction scores were recorded under bright-field microscope. At least 10 randomly selected fields (10 × ) from each mouse and four mice per genotype were analysed. (Data are shown as mean±s.e.m.,Pvalues are indicated on the figures. Ductular reaction scores, unpaired Student’st-test; necrotic foci, Mann–WhitneyU-test,n=4 mice each group). BD, bile duct; CV, central vein; PV, portal vein. Figure 5: NRBF2 KO mice have no enhanced mortality but with focal liver nercrosis. ( a ) The gross anatomical views of representative 4% paraformaldehyde-fixed livers and quantification of liver index. (Data are shown as mean±s.e.m., P values are indicated on the figures, unpaired Student’s t -test, n =3 mice each group). Scale bar, 1 cm. ( b ) The haematoxylin and eosin (H&E) and CD45 staining of 10-month-old WT and NRBF2 KO mice livers. The NRBF2 KO liver shows mild increase of ductular reaction (yellow arrow) and isolated necrosis (red arrows). The necrotic foci were further confirmed by CD45 staining (black arrow). This is a representative image from four mice per genotype. Scale bar, 50 μm. ( c ) The number of necrotic foci and ductular reaction scores were recorded under bright-field microscope. At least 10 randomly selected fields (10 × ) from each mouse and four mice per genotype were analysed. (Data are shown as mean±s.e.m., P values are indicated on the figures. Ductular reaction scores, unpaired Student’s t -test; necrotic foci, Mann–Whitney U -test, n =4 mice each group). BD, bile duct; CV, central vein; PV, portal vein. Full size image Abnormal Vps34 activity and Nrf2 pathway in NRBF2 KO liver Examination of autophagy and ubiquitin proteasome system substrates indicated increased levels of p62 ( Fig. 6a,b ) and ubiquitin-positive protein species with high-molecular weight ( Fig. 6c ) in the lysates of NRBF2 KO liver. Also, the levels of Atg14L-linked Vps34 activity are remarkably reduced in the mutant liver ( Fig. 6d,e ). Interestingly, immunofluorescence staining revealed accumulation of p62 in many hepatocytes that appear clustered in NRBF2 KO livers ( Fig. 6f ). These p62-positive hepatocytes are also labelled with antibodies against ubiquitin ( Supplementary Fig. 5c ) and NAD(P)H dehydrogenase, quinone 1 (NQO1) ( Fig. 6g ), the antioxidant enzyme under the control of transcription factor Nrf2, suggesting the activation of Nrf2 pathway [21] . Furthermore, we found extensive staining of the apoptotic marker cleaved caspase-8 ( Supplementary Fig. 5d ) in isolated hepatocytes in the mutant liver; cleaved caspase-8 signal overlaps with p62 accumulation. The accumulation of p62 in some but not all hepatocytes suggests that NRBF2 deficiency only partially impairs autophagic activity in the liver. In addition, lack of NRBF2 may result in sporadic apoptosis of hepatocytes. 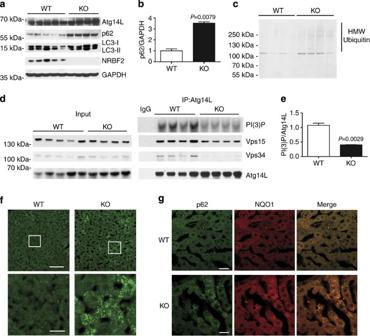Figure 6: NRBF2 KO livers display reduced Atg14L-linked Vps34 activity, partially impaired autophagy and focal activation of Nrf2 pathway. (a) WB analysis shows accumulation of p62 in the liver of NRBF2 KO mice. Liver lysates were immunoprobed with antibodies indicated. p62 protein levels are upregulated in the KO mice liver. (b) The quantification result shows that the p62 level increased more than threefold in the NRBF2 KO mice liver compared with WT mice liver. (Data are shown as mean±s.e.m.,Pvalues are indicated on the figures, unpaired Student’st-test; WT,n=5 mice; KO,n=4 mice). (c) WB analysis shows accumulation of high-molecular weight (HMW) ubiqutin in the liver of NRBF2 KO mice. Insoluble fractions of liver lysates were immunoprobed with an anti-ubiquitin antibody,n=4 mice per genotype. (d) Atg14L-linked Vps34 kinase activity is impaired in the liver of NRBF2 KO mice. Atg14L-linked Vps34 is pulled down by an anti-Atg14L antibody and is subjected to KA. IP products and inputs were immunoblotted using the antibodies indicated. (e) Quantification of IPed Vps34 kinase activity versus IPed Atg14L shows the significant difference between WT and NRBF2 KO mice liver. (Data are shown as mean±s.e.m.,Pvalues are indicated on the figure, unpaired Student’st-test,n=4 mice each group). (f) Focal accumulation of p62 in the liver of NRBF2 KO mice. Liver frozen sections (15 μm in thickness) were stained with an anti-p62 antibody. Focal accumulation of p62 is observed in the KO mice liver but not in the WT mice liver. Scale bars, 100 μm or 20 μm (amplified regions). This is a representative image from four mice per genotype. (g) Accumulated p62 colocalizes with NQO1. Liver frozen sections were double stained with an anti-p62 antibody and an anti-NQO1 antibody. This is a representative image from four mice per genotype. Scale bars, 20 μm. Figure 6: NRBF2 KO livers display reduced Atg14L-linked Vps34 activity, partially impaired autophagy and focal activation of Nrf2 pathway. ( a ) WB analysis shows accumulation of p62 in the liver of NRBF2 KO mice. Liver lysates were immunoprobed with antibodies indicated. p62 protein levels are upregulated in the KO mice liver. ( b ) The quantification result shows that the p62 level increased more than threefold in the NRBF2 KO mice liver compared with WT mice liver. (Data are shown as mean±s.e.m., P values are indicated on the figures, unpaired Student’s t -test; WT, n =5 mice; KO, n =4 mice). ( c ) WB analysis shows accumulation of high-molecular weight (HMW) ubiqutin in the liver of NRBF2 KO mice. Insoluble fractions of liver lysates were immunoprobed with an anti-ubiquitin antibody, n =4 mice per genotype. ( d ) Atg14L-linked Vps34 kinase activity is impaired in the liver of NRBF2 KO mice. Atg14L-linked Vps34 is pulled down by an anti-Atg14L antibody and is subjected to KA. IP products and inputs were immunoblotted using the antibodies indicated. ( e ) Quantification of IPed Vps34 kinase activity versus IPed Atg14L shows the significant difference between WT and NRBF2 KO mice liver. (Data are shown as mean±s.e.m., P values are indicated on the figure, unpaired Student’s t -test, n =4 mice each group). ( f ) Focal accumulation of p62 in the liver of NRBF2 KO mice. Liver frozen sections (15 μm in thickness) were stained with an anti-p62 antibody. Focal accumulation of p62 is observed in the KO mice liver but not in the WT mice liver. Scale bars, 100 μm or 20 μm (amplified regions). This is a representative image from four mice per genotype. ( g ) Accumulated p62 colocalizes with NQO1. Liver frozen sections were double stained with an anti-p62 antibody and an anti-NQO1 antibody. This is a representative image from four mice per genotype. Scale bars, 20 μm. Full size image Loss of NRBF2 enhances cell vulnerability to ER stress To characterize NRBF2 physiological function, we treated WT and NRBF2 KO MEFs with ER stress inducers thapsigargin or tunicamycin, and analysed cell fate. The KO MEFs are apparently more vulnerable to ER stress than WT MEFs as shown with cell morphology changes ( Fig. 7a ) and cell death increase (by propidium iodide staining; Fig. 7b ). The vulnerability of NRBF2 KO MEFs to ER stress can be reversed by re-introducing CFP-tagged NRBF2 ( Fig. 7c ), indicating rescue of defective NRBF2 KO MEFs and strengthening the role for NRBF2 in preventing ER stress-induced cytotoxicity. We next examined ER stress markers (Bip and Chop), p62, LC3 and apoptotic markers (cleaved Caspase-8 and -3) in treated cells. Compared with WT MEFs, KO MEFs showed similar levels of induced ER stress markers, but clearly impaired autophagy activation and enhanced apoptosis at 24 h post treatment ( Fig. 7d ). Although no obvious differences were observed in the levels of full-length caspase-8 between WT and KO MEFs, cleaved caspase-8 (p18 and p43) accumulated in the KO MEFs, suggesting impaired degradation of cleaved caspase-8 rather than enhanced cleavage of caspase-8 in the NRBF2 KO MEFs after ER stress induction. In addition, we found co-localization of p62 and cleaved capase-8 within accumulated foci in thapsigargin-treated NRBF2 KO MEFs ( Fig. 7e ). 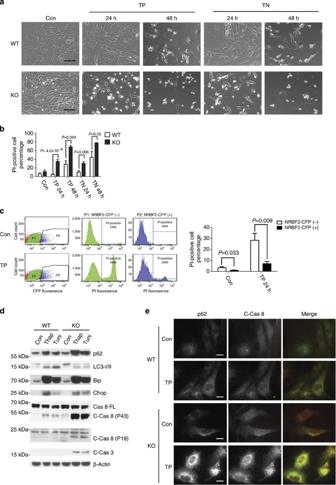Figure 7: Loss of NRBF2 enhances the vulnerability of the cells to ER stress. WT and NRBF2 KO MEFs were treated with DMSO, 1 μM thapsigargin (TP) or 1 μM tunicamycin (TN) for 24 or 48 h. (a) Then cells were either imaged under phase-contrast microscope or (b) stained with propidium iodide (PI) and subjected to cell death rate analysis by flow cytometry. The representative images of cell morphology after treatments and quantitative analysis of PI-positive cells rate show marked increase of cell death in the NRBF2 KO MEFs compared with WT MEFs. (Data are shown as mean±s.e.m.,Pvalues are indicated on the figure, unpaired Student’st-test,n=5). Scale bars, 100 μm; Con, control. (c) Re-introducing NRBF2 to NRBF2 KO MEFs reverses the vulnerability of cells to ER stress. NRBF2-CFP stably expressing cells were established in the NRBF2 KO background. Cells were treated with DMSO or 1 μM TP for 24 h then stained with PI and subjected to cell death rate analysis by flow cytometry. The cell death rate in CFP-positive (+) population (NRBF2-CFP expression) and negative (−) population (no NRBF2-CFP expression) were recorded and analysed, respectively. (Data are shown as mean±s.e.m.,Pvalues are indicated on the figure, unpaired Student’st-test,n=3). (d) ER stress inducers trigger caspase-8 and caspase-3 activation in NRBF2 KO MEFs. MEFs were treated with DMSO, 1 μM TP or 1 μM TN for 24 h, and then immunoprobed with indicated antibodies. Marked accumulation of cleaved caspase-8 (C-Cas 8; p43 and p18 units) and cleaved caspase-3 (C-Cas 3) are observed in the NRBF2 KO MEFs but not WT MEFs treated with TP or TN. This is a representative image from three independent experiments. (e) C-Cas 8 preferentially localizes at p62 aggregation foci. MEFs were treated with DMSO or 1 μM TP for 24 h, and then co-stained with an anti-p62 antibody and an anti-cleaved caspase-8 antibody. The C-Cas 8 fluorescence signals are triggered in NRBF2 KO MEFs treated with TP and preferentially localize at p62 aggregation foci. Scale bars, 20 μm. This is a representative image from three independent experiments. Figure 7: Loss of NRBF2 enhances the vulnerability of the cells to ER stress. WT and NRBF2 KO MEFs were treated with DMSO, 1 μM thapsigargin (TP) or 1 μM tunicamycin (TN) for 24 or 48 h. ( a ) Then cells were either imaged under phase-contrast microscope or ( b ) stained with propidium iodide (PI) and subjected to cell death rate analysis by flow cytometry. The representative images of cell morphology after treatments and quantitative analysis of PI-positive cells rate show marked increase of cell death in the NRBF2 KO MEFs compared with WT MEFs. (Data are shown as mean±s.e.m., P values are indicated on the figure, unpaired Student’s t -test, n =5). Scale bars, 100 μm; Con, control. ( c ) Re-introducing NRBF2 to NRBF2 KO MEFs reverses the vulnerability of cells to ER stress. NRBF2-CFP stably expressing cells were established in the NRBF2 KO background. Cells were treated with DMSO or 1 μM TP for 24 h then stained with PI and subjected to cell death rate analysis by flow cytometry. The cell death rate in CFP-positive (+) population (NRBF2-CFP expression) and negative (−) population (no NRBF2-CFP expression) were recorded and analysed, respectively. (Data are shown as mean±s.e.m., P values are indicated on the figure, unpaired Student’s t -test, n =3). ( d ) ER stress inducers trigger caspase-8 and caspase-3 activation in NRBF2 KO MEFs. MEFs were treated with DMSO, 1 μM TP or 1 μM TN for 24 h, and then immunoprobed with indicated antibodies. Marked accumulation of cleaved caspase-8 (C-Cas 8; p43 and p18 units) and cleaved caspase-3 (C-Cas 3) are observed in the NRBF2 KO MEFs but not WT MEFs treated with TP or TN. This is a representative image from three independent experiments. ( e ) C-Cas 8 preferentially localizes at p62 aggregation foci. MEFs were treated with DMSO or 1 μM TP for 24 h, and then co-stained with an anti-p62 antibody and an anti-cleaved caspase-8 antibody. The C-Cas 8 fluorescence signals are triggered in NRBF2 KO MEFs treated with TP and preferentially localize at p62 aggregation foci. Scale bars, 20 μm. This is a representative image from three independent experiments. Full size image NRBF2 stabilizes Vps34-Vps15-Beclin1-Atg14L complex in vivo Although NRBF2 is important for Atg14L’s interaction with Beclin 1, Vps34 and Vps15 proteins in MEFs ( Fig. 2 ), it is unclear whether NRBF2 affects differential Vps34 complex formation particularly in tissues. We performed western blotting (WB) to examine the total protein levels of Vps34, Vps15, Beclin 1, UVRAG and Atg14L in NRBF2 WT and KO mice brain lysates. We found little change in basal protein levels between NRBF2 WT and KO mice ( Fig. 8a ). However, using anti-Vps34 antibody to pull down Vps34 protein complexes, we found that Vps34 binds markedly less Atg14L in NRBF2 KO MEFs (~75% decrease compared to WT mice). Vps34 also binds less Vps15 (~35% reduced) and Beclin 1 (~40% reduced) in KO mice. In contrast, Vps34-associated UVRAG are similar between NRBF2 WT and KO mice. Measurement of the activity of Vps34 IP product shows a decrease in PI(3)P production in NRBF2 KO mice ( Fig. 8a,b ). This result provides strong evidence that NRBF2 is required for an activated Vps34 activity by stabilizing the Vps34-Vps15-Beclin 1-Atg14L complex formation. 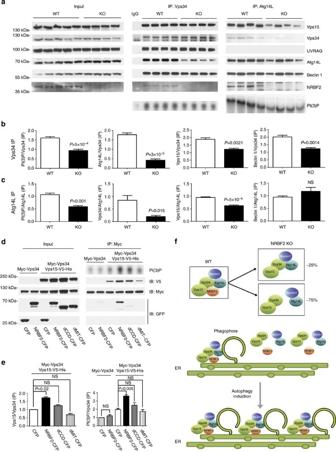Figure 8: Assembly of Beclin 1-Vps34 complex in WT and NRBF2 KO mice and schematic model for the NRBF2 function. (a) NRBF2 is critical for the assembly of Vps34-Vps15 and Atg14L-Beclin 1 complex. Brain lysate from WT and NRBF2 KO mice were subjected to co-IP by Vps34 antibody and Atg14L antibody. The IP products were subjected toin vitrolipid KA and WB analysis using the indicated antibodies. (b,c) Quantification results shows that Vps34-Vps15 and Atg14L-Beclin 1 complex interactions as well as Atg14L-linked Vps34 kinase activity are markedly impaired in NRBF2 KO mice. (Data are shown as mean±s.e.m.,Pvalues are indicated on the figures, unpaired Student’st-test,n=4 mice in each group; NS, not significant). (d) Overexpression of NRBF2 enhances overall Vps34 kinase activity. HEK293T cells were co-transfected with Myc-Vps34-Vps15-His and CFP, NRBF2-CFP, dMIT-CFP or dCCD-CFP. Total Vps34 was pulled down by an anti-myc antibody and subjected to KA. IP products and inputs are immunoblotted using the antibodies indicated. (e) Quantification of IPed Vps34 kinase activity, Vps15 protein normalized with IPed Vps34 shows that NRBF2-CFP, but not CFP, dMIT-CFP or dCCD-CFP significantly enhance Vps34 kinase activity and Vps34-Vps15 interaction. (Data are shown as mean±s.e.m.,Pvalues are indicated on the figures. IPed Vps15/IPed Vps34, one samplet-test versus hypothetical mean 1, Bonferroni correction,n=3; IPed Vps34 kinase activity/IPed Vps34, multiplet-test followed by Bonferroni correction,n=3). (f) Schematic model for the NRBF2 function in autophagy. Top: in WT cells, NRBF2 functions to stabilize Beclin 1-Atg14L, Vps34 and Vps15 proteins in the specific autophagy PI3K-III kinase complex. In NRBF2 KO cells, ~25% Atg14L remains in the complex with Vps34-Vps15; middle and bottom: upon autophagy induction, NRBF2-Atg14L interaction mediates the binding with other components in the cytosol and consequent assembly of a highly active PI3K-III kinase complex at the phagophore, resulting in enhanced autophagy capacity. Figure 8: Assembly of Beclin 1-Vps34 complex in WT and NRBF2 KO mice and schematic model for the NRBF2 function. ( a ) NRBF2 is critical for the assembly of Vps34-Vps15 and Atg14L-Beclin 1 complex. Brain lysate from WT and NRBF2 KO mice were subjected to co-IP by Vps34 antibody and Atg14L antibody. The IP products were subjected to in vitro lipid KA and WB analysis using the indicated antibodies. ( b , c ) Quantification results shows that Vps34-Vps15 and Atg14L-Beclin 1 complex interactions as well as Atg14L-linked Vps34 kinase activity are markedly impaired in NRBF2 KO mice. (Data are shown as mean±s.e.m., P values are indicated on the figures, unpaired Student’s t -test, n =4 mice in each group; NS, not significant). ( d ) Overexpression of NRBF2 enhances overall Vps34 kinase activity. HEK293T cells were co-transfected with Myc-Vps34-Vps15-His and CFP, NRBF2-CFP, dMIT-CFP or dCCD-CFP. Total Vps34 was pulled down by an anti-myc antibody and subjected to KA. IP products and inputs are immunoblotted using the antibodies indicated. ( e ) Quantification of IPed Vps34 kinase activity, Vps15 protein normalized with IPed Vps34 shows that NRBF2-CFP, but not CFP, dMIT-CFP or dCCD-CFP significantly enhance Vps34 kinase activity and Vps34-Vps15 interaction. (Data are shown as mean±s.e.m., P values are indicated on the figures. IPed Vps15/IPed Vps34, one sample t -test versus hypothetical mean 1, Bonferroni correction, n =3; IPed Vps34 kinase activity/IPed Vps34, multiple t -test followed by Bonferroni correction, n =3). ( f ) Schematic model for the NRBF2 function in autophagy. Top: in WT cells, NRBF2 functions to stabilize Beclin 1-Atg14L, Vps34 and Vps15 proteins in the specific autophagy PI3K-III kinase complex. In NRBF2 KO cells, ~25% Atg14L remains in the complex with Vps34-Vps15; middle and bottom: upon autophagy induction, NRBF2-Atg14L interaction mediates the binding with other components in the cytosol and consequent assembly of a highly active PI3K-III kinase complex at the phagophore, resulting in enhanced autophagy capacity. Full size image Consistent with our in vitro data ( Fig. 2a ), anti-Atg14L IP product from NRBF2 KO brain lysates showed reduced levels of Vps15, Vps34 proteins and Vps34 kinase activity (PI(3)P production) but unaltered Beclin 1 protein level, compared with WT lysates ( Fig. 8a,c ). This result suggests that NRBF2 has little effect on Beclin 1-Atg14L complex formation, but has a role in Vps34-Vps15-Beclin 1-Atg14L complex assembly by bringing Vps15 and Atg14L-bound Beclin 1 to Vps34. To evaluate the role of Vps15 in this context, we co-expressed NRBF2-CFP and Myc-Vps34 with or without Vps15-V5-His in HEK293T cells, IPed the transfected cell lysates with anti-Myc antibody and measured PI(3)P production. The results show that NRBF2-CFP expression has no effect on Vps34 activity in the absence of Vps15-V5-His. In contrast, in the presence of Vps15-V5-His, NRBF2-CFP expression drastically enhances the Vps34 kinase activity when compared with CFP control ( Fig. 8d,e ) suggesting that Vps15 is required for NRBF2’s effect on Vps34 kinase activity. Interestingly, we found that both the MIT domain and CCD are important for the function of NRBF2 in enhancing Vps15-mediated Vps34 activity under these conditions ( Fig. 8d,e ). It is worth mentioning that, distinct from GFP-tagged Beclin 1, Atg14L, UVRAG or Rubicon, overexpression of NRBF2-CFP causes enhanced Vps34 activity when co-expressing Myc-Vps34 and Vps15-His in HEK293T cells ( Supplementary Fig. 6 ). Taken together, our data suggest a critical role for NRBF2 in assembling specific PI3K-III complex by recruiting the subcomplex Beclin 1-Atg14L and Vps15 to Vps34, creating a highly active PI3K-III kinase complex. Our study identifies NRBF2 as a new component in the Beclin 1-Vps34 complex and a critical modulator of PI3K-III activity in autophagy regulation. Thus, it adds a new member to the growing list of Beclin 1-Vps34-binding partners that regulate cellular functions of PI3K-III. Previous studies reported NRBF2 within the network of the human autophagy system [22] and in the association with SCOC, a Golgi protein involved in starvation-induced autophagy [23] , thereby hinting at its role in autophagy. But the exact function of NRBF2 in autophagy remains uncharacterized. Our study not only reveals the function of NRBF2 in autophagy regulation, but also demonstrates its role in suppressing ER stress-induced apoptotic death and liver necrosis. Beclin 1-Vps34-Vps15 is the conserved core component of PI3K-III complex that binds either Atg14L or UVRAG tightly, and thus forms multiple stable PI3K-III complexes. These stable complexes are the essential functional units that dictate various cellular functions of PI3K-III (ref. 10 ). Our identification of NRBF2 through two independent affinity purification procedures ( Fig. 1a,g ) suggests that NRBF2 is also a stable constituent in the Beclin 1-Vps34 complex. Our data demonstrate that NRBF2 directly binds Atg14L to associate with Beclin 1, Vps34 and Vps15 proteins, and modulates Atg14L-linked Vps34 kinase activity. Thus, we conclude that NRBF2 is an integral part of the Atg14L-associated PI3K-III complex that has a role in autophagy initiation. While this manuscript was in revision, a report showed that the yeast protein Atg38, which shares sequence homology to NRBF2, binds yeast Atg14 and regulates Vps34 activity via its MIT domain [24] . Thus, our study demonstrates that NRBF2 is mammalian homologue of yeast Atg38, and the function of Atg38/NRBF2 in controlling Atg14L-linked Vps34 kinase activity is evolutionarily conserved. Our study provides insight into the mechanism whereby NRBF2 modulates specific PI3K-III kinase complex activity in vivo . Our data suggest that NRBF2 has a critical role in assembling the Vps34-Vps15-Beclin 1-Atg14L complex by linking the subcomplex Beclin 1-Atg14L and Vps15 to the catalytic subunit Vps34 in tissues for a highly functional PI3K-III kinase complex ( Fig. 8e ). We notice that NRBF2 is neither important for Beclin 1-Atg14L subcomplex formation nor critical for UVRAG binding to Vps34. In contrast, NRBF2 is crucial for the Vps15-Vps34 stable interaction and optimal Vps34 lipid kinase activity [25] . This evidence suggests that NRBF2 may modulate Vps15-mediated Vps34 activity independent of Atg14L. Indeed, unlike Atg14L, NRBF2 seems to interact with UVRAG, a component in a distinct Beclin 1-Vps34 complex exclusive of Atg14L, although the binding is weaker compared with NRBF2’s binding to Atg14L ( Fig. 1c,g ). UVRAG-linked Vps34 activity is known to regulate autophagy maturation [12] , [18] . Interestingly, we find that NRBF2-deficient MEFs have a reduced number of mature autophagosomes, suggesting the involvement of NRBF2 in autophagy maturation. Consistently, increased NRBF2 levels facilitate UVRAG-linked Vps34 kinase activity. Therefore, our data suggest that NRBF2 is a distinct modulator of Vps34 activity throughout the autophagy process. The characterization of NRBF2 KO mice clearly shows that Nrbf2 is not an essential gene. Indeed, no mortality is observed in NRBF2 KO mice for at least 12 months and they appear largely normal. The observation is in contrast to that of KO mice for Vps34 (ref. 14 ), Beclin 1 (ref. 13 ) or Atg14L (our unpublished data), each of which is embryonic lethal. Furthermore, ablation of genes for autophagy conjugation components, such as Atg3 , Atg5 or Atg7 , causes perinatal death in mice [26] , [27] , [28] , indicating a developmental role of autophagy. Conditional deletion of autophagy-related genes in a tissue-specific manner shows severe pathologies in the liver, including hepatomegaly, hepatic steatosis, liver tumours and oxidative stress [16] , [29] , [30] . Interestingly, despite impaired Atg14L-linked Vps34 activity and turnover of the autophagic substrate p62 (for example, in the liver), NRBF2 KO mice are spared of obvious developmental blocks and they survive normally. Therefore, it is likely that NRBF2 KO mice retain some autophagic activity. Indeed, our study demonstrates that Atg14L-linked Vps34 protein levels and lipid kinase activity were reduced by 75% in NRBF2 KO tissues. The remaining 25% activity of the Atg14L-Vps34 kinase complex is perhaps able to sustain basal requirement of autophagy function in many cells or tissues. This notion is also supported by the fact that NRBF2 KO livers show mild lesions associated with focal necrosis, inflammation, isolated apoptotic hepatocytes and activated Nrf2 pathway. Thus, it is unlikely that NRBF2 has an essential role in basal autophagy, particularly under normal conditions. We conclude that NRBF2 is a key factor for modulating the capacity of Vps34 activity in response to various stresses that induce autophagy. Finally, our data reveal an important function of NRBF2 in protecting cells from ER stress-induced cell death, consistent with its significant role in condition-specific autophagy modulation rather than in basal autophagy regulation. The result may implicate NRBF2 in the regulation of biochemical activity or cellular function of p62, which is a multifaceted adaptor protein for an array of cellular processes, including the ubiquitin proteasome system, autophagy and apoptosis [31] , [32] . In summary, our study identifies NRBF2 as a key modulator of PI3K-III activity by stabilizing Beclin 1, Atg14L, Vps34 and Vps15 proteins in the assembly of highly active PI3K-III kinase complexes. NRBF2 has an important role in autophagy control particularly under stress. NRBF2 KO mice thus provide a valuable tool for future studies to dissect the physiological functions of PI3K-III in vivo under normal as well as human disease conditions. Reagents and antibodies Dynabeads protein G, anti-Myc affinity gel beads, NuPAGE Bis-Tris gels, MES and MOPS SDS running buffer, Lipofectamine 2000 and Lipofectamine RNAi MAX kits, Atg14L siRNA, 4′,6-diamidino-2-phenylindole (DAPI)-containing fluorescence mounting medium and propidium iodide were purchased from Invitrogen (Carlsbad, CA, USA). EDTA-free protease inhibitor cocktail tablets and phosphatase inhibitor cocktail tablets were purchased from Roche Diagnostics (Indianapolis, IN, USA). Hybond-P polyvinylidene difluoride (PVDF) membrane was purchased from GE Healthcare Life Sciences (Pittsburgh, PA, USA). BCA Protein Assay Reagent Kit was purchased from Pierce (Rockford, IL, USA). Tunicamycin and thapsigargin were purchased from Calbiochem (La Jolla, CA, USA). Gel filtration calibrant mixtures were purchased from Bio-Rad (Hercules, CA, USA). Radioactive 32 P-ATP and 3 H-leucine were purchased from PerkinElmer (Waltham, MA, USA). Mouse monoclonal M2 FLAG affinity gel beads, anti-HA affinity gel beads and G418 and phosphatidylinositol were purchased from Sigma (St Louis, MO, USA). NRBF2 siRNA were purchased from Dharmacon (Lafayette, CO, USA). Sequencing grade trypsin was purchased from Promega (Fitchburg, WI, USA). Coated silica gel was purchased from Whatman (Kent, UK). Optimal cutting temperature embedding medium was purchased from Sakura finetek USA (Torrance, CA, USA). Anti-NRBF2 (cat. no. 8633 for WB, 1:500), LC3B (Cat. no. 2775 for WB, 1:1,000), UVRAG (cat. no. 5320, 1:1,000), BiP (cat. no. 3177, 1:1,000), CHOP (cat. no. 2895, 1:1,000), Myc (cat. no. 2276, 1:1,000), FLAG (cat. no. 2368, 1:1,000), β-actin (cat. no. 3700, 1:5,000), cleaved capsase-8 (cat. no. 8592 for WB, 1:1,000; and immunostaining, 1:800) and cleaved caspase-3 (cat. no. 9661, 1:1,000) antibodies were purchased from Cell Signaling Technology. Anti-NRBF2 antibody (cat. no. A301-852A for IP, 1:100) was purchased from Bethyl Laboratories (Montgomery, TX, USA). Anti-Vps34 antibody for WB (cat. no. 38-2100, 1:1,000) was purchased from Invitrogen. Anti-Vps34 antibody for IP (cat. no. Z-R015, 1:100) was purchased from Echelon Biosciences (Salt Lake City, UT, USA). Anti-Atg14L (cat. no. PD026, WB 1:1,000; IP 1:100) and LC3B (cat. no. PM036 for immunostaining, 1:2,000) antibodies were obtained from MBL. Anti-WIPI2 (cat. no. 101985, 1:300) and NQO1 (cat. no. ab2346, 1:500) antibodies were purchased from Abcam (Cambridge, MA, USA). Anti-Beclin 1 antibody (cat. no. sc-11427, 1:1,000) was purchased from Santa Cruz Biotechnology (Santa Cruz, CA, USA). Anti-p62/SQSTM1 antibody (cat. no. 03-GP62-C, WB 1:1,000; immunostaining 1:1,000) was purchased from American Research Products, Inc. (Belmont, MA, USA). Anti-GFP antibody (cat. no. 11814460001, 1:1,000) was purchased from Roche Diagnostics. Anti-caspase-8 antibody (cat. no. AF1650 for WB, 1:1,000) was purchased from R&D Systems (Minneapolis, MN, USA). Anti-ubiquitin antibody (cat. no. Z0458, WB 1:1,000; immunostaining 1:300) was purchased from Dako (Carpinteria, CA, USA). Fluorescence-conjugated secondary antibodies for immunostaining (1:500) were purchased from Invitrogen. NRBF2 interactome proteomic analysis Sequence-validated ORF encoding for NRBF2 in pDONR223 were recombined into the Gateway destination vectors MSCV-Tet-FLAG-HA-IRES-PURO (which uses a tetracycline-inducible cytomegalovirus (CMV) promoter; iTAP) for generation of a stable cell line using λ recombinase. Virus was produced for indicated ORFs by co-transfecting the respective iTAP, GAG/POL and VSVG plasmids into 293T cells. After packaging, viruses were used to infect TREx-293 (Invitrogen) cells and subsequently selected for stable expression using 1 μg ml −1 puromycin. About 1 × 10 7 cells stably expressing N-terminally HA-tagged NRBF2 were harvested and lysed with 3 ml lysis buffer (50 mM Tris, pH 7.5, 150 mM NaCl, 0.5% Nonidet P40 (NP40) and EDTA-free protease inhibitor cocktail tablets). Centrifugation-cleared lysates (13,000 r.p.m.) were filtered through 0.45 mm spin filters (Millipore Ultrafree-CL) and immunoprecipitated with 60 μl anti-HA resin. Resin containing immune complexes was washed five times with lysis buffer followed by five PBS washes, and elution with 150 μl of 250 mg ml −1 HA peptide in PBS. Eluted immune complexes were precipitated with 20% trichloroacetic acid (TCA) and pellets were washed once with 10% TCA and four times with cold acetone. Precipitated proteins were resuspended in 50 mM ammonium bicarbonate (pH 8.0) with 20% acetonitrile and incubated with sequencing grade trypsin at a concentration of 12.5 ng ml −1 at 37 °C for 4 h. Trypsin reactions were quenched by addition of 5% formic acid and peptides were desalted using C18 Stage Tips. For each Liquid chromatography coupled to tandem mass spectrometry run using an LTQ Velos linear ion trap mass spectrometer (Thermo Scientific), 4 μl were loaded onto a 18 cm × 125 μm (ID) C18 column and peptides eluted using a 50-min 8–26% acetonitrile gradient. Spectra were acquired using a data-dependent Top-10 method. Each sample was shot twice in succession, followed by a wash with 70% acetonitrile and 30% isopropanol. Tandem MS/MS data were searched using Sequest and a concatenated target-decoy uniprot human database with a 2-Da mass window. All data were filtered to a 1% false discovery rate (peptide level) before analysis using CompPASS [33] . Gel filtration Mouse brain was homogenized in two volumes of ice-cold homogenization buffer (0.32 M sucrose, 1 mM NaHCO 3 , 20 mM HEPES (pH 7.4), 0.25 mM CaCl 2, 1 mM MgCl 2 , 100 μM PMSF, 1 μg ml −1 Pepstain and protease inhibitor cocktail). Brain extracts were diluted with equal volumes of 2 × pull-out buffer (1 × pull-out buffer containing 20 mM HEPES, pH 7.4, 1 mM MgCl 2 , 0.2% Triton X-100, 150 mM NaCl 100 μg ml −1 PMSF, 2 μg ml −1 Pepstain and protease inhibitor cocktail) and incubated for 15 min at 4 °C. The homogenate was subjected to low-speed centrifugation at 21,000 g for 10 min. The resulting supernatant was then applied to a Superdex 200 HR 10/30 column (GE Healthcare Biosciences) and eluted at a flow rate of 0.5 ml min −1 . Fractions (0.25 ml) were examined by WB. Generation and genotyping of NRBF2 KO mice Embryonic stem cells with Nrbf2 gene disruption (Ayu21-W143) has been obtained by gene trap method. The trap vector is pU-21W. The insertion site of trap vector is located at the first intron of Nrbf2 gene (at 4,767–4,768), confirmed by DNA sequencing. Nrbf2 gt/+ embryonic stem cells were used to generate chimaeric mice using the aggregation method. Heterozygous mutant mice were outbred with C57BL/6 mice and interbred to obtain homozygous mutant mice. Genotyping of NRBF2 mice were executed by PCR with forward primer (primer F: 5′-GACAGCTATATCAGGGTCCTG-3′) and reverse primers (primer R1 for Nrbf2 genome; 5′-GATCAAGCAGTACCTCCAAAC-3′; primer R2 for pU-21W; 5′-CCGGCTAAAACTTGAG ACCTTC-3′). WT band is 339 bp, mutant band is 488 bp. Generation of WT and NRBF2 KO stable cell lines NRBF2 WT and KO embryos were generated from cross-breeding Nrbf2 gt/+ mice. Embryonic fibroblasts were prepared from 12.5 day embryos. Once the genotype of the embryos were confirmed by PCR, the mouse embryonic fibroblasts cells were transformed with an SV40 large T antigen expression vector, and immortalized cell lines were established. Cell culture Human embryonic kidney cell line HEK293T, MEF cell line NIH3T3 and MEFs were maintained in Dulbecco’s modified Eagle’s medium (DMEM, Invitrogen) supplemented with 10% fetal bovine serum (Invitrogen) and 50 μg ml −1 penicillin and streptomycin (Invitrogen). Transient DNA transfection of HEK293T and MEF cells was performed using Lipofectamine 2000 kit according to the manufacturer’s manual (Invitrogen). Transfection of siRNA into NIH3T3 cells was performed using Lipofectamine RNAi MAX kit following manufacturer’s reverse transfection protocol (Invitrogen). Animal tissue samples preparation All animal study protocols were approved by the institutional animal welfare committee of the Icahn School of Medicine at Mount Sinai. Mice were transcardic perfused with ice-cold PBS to remove excessive blood. For WB and Vps34 in vitro KA, liver tissues were dissected and homogenized in RIPA buffer (50mM Tris-HCl, pH 7.5, 1% NP40, 0.35% DOC, 150 mM NaCl, 1 mM EDTA, 1 mM EGTA, supplemented with protease and phosphatase inhibitor cocktails) or IP lysis buffer (10 mM Tris-HCl, pH 7.5, 2 mM EDTA, 1% NP40, 150 mM NaCl, supplemented with protease and phosphates inhibitor cocktail). The tissues homogenates were centrifuged at 1,000 g for 10 min to remove nucleus and pellets. The supernatants were collected and saved at −80 °C for further analysis. For histology examination, liver tissues were dissected and fixed in 4% PFA/PBS overnight. Fixed liver blocks then were either embedded with paraffin for haematoxylin and eosin staining or dehydrated in 30% sucrose before optimal cutting temperature medium embedding for immunostaining. Immunostaining and microscopy Fixed cells or tissue sections were permeablized in 0.2% Triton X-100/PBS for 10–30 min at room temperature. After blocking in 5% goat serum/0.2% Triton X-100/PBS for 30 min at room temperature, cells or tissue sections were incubated in primary antibodies overnight at 4 °C. After three washes with PBS, cells or tissue sections were incubated with fluorescence-conjugated secondary antibodies for 1 h at room temperature. After three washes with PBS, cells or tissue sections were mounted with fluorescence mounting medium and examined under Olympus IX70 (Tokyo, Japan) fluorescent microscope or Zeiss CLSM 780 (Göttingen, Germany) confocal microscope. WB and IP For WB analysis, cells or tissues were homogenized and lysed in RIPA buffer. Lysates were denature in 1 × Laemmli sample buffer and resolved by SDS-PAGE. For IP, cells or tissues were homogenized and lysed in IP lysis buffer. Lysates were incubated with antibodies overnight and followed by 1 h incubation with Dynabeads protein G (Atg14L antibody IP), or incubated with antibody affinity gel beads overnight (FLAG and Myc antibodies IP). Beads were washed five times with IP lysis buffer and denatured in 1 × Laemmli sample buffer before resolving by SDS-PAGE. The full scans of critical western blots are provided in the Supplementary Fig. 7 . In vitro Vps34 lipid KA : In vitro Vps34 lipid KA was performed as previously described with minor modification [18] . In brief, Vps34 immune-complex beads were washed once with KA buffer (20 mM HEPES, pH 7.4, 1 mM EGTA, 0.4 mM EDTA and 5 mM MgCl 2 ), then suspended in 50 μl KA buffer containing 50 μM cold ATP, 5 mM MnCl 2 , 50 μM DTT, 0.1 mg ml −1 sonicated phosphatidylinositol and 5 μCi 32 P-ATP. The mixtures were incubated at 37 °C for 30 min with vigorous shaking. The reactions were stopped by adding 120 μl of CHCl3/CH3OH/HCl (10:20:0.2) followed by vigorous shaking for 5 min. The organic phase (lower phase) was separated by centrifuging for 5 min and 15 μl of the organic phase was spotted onto a silica gel thin-layer plate followed by chromatography separation for 30 min in CHCl 3 /CH 3 OH/NH 4 OH/H 2 O (86:76:10:14). 32 P-PI(3)P radioactivity was recorded with Typhoon 9,400 Variable Imager (GE Healthcare Biosciences, Little Chalfont, UK). Long-lived protein degradation assay Long-lived protein degradation was measured as described previously [34] . In brief, NIH3T3 cells were transfected with either control or Atg14L or Nrbf2 SiRNA and plated in 12-well plates, respectively. After 48 h, DMEM was changed to leucine-free medium supplemented with 1 μCi ml −1 3 H-leucine adjusted to 62.4 μM and incubated at 37 °C, 5% CO 2 . After being pulse-labelled for 24 h, cells were washed three times and cultured in DMEM supplemented with excess unlabelled leucine (5 mM) for 16 h to chase out short-lived proteins. Cells were then washed three times and further cultured for 4 h in DMEM, Earle’s Balanced Salt Solution or Earle’s Balanced Salt Solution supplemented with 100 nM Wortmannin, all containing unlabelled leucine (5 mM). Both medium and cell lysates were subject to TCA precipitation. Long-lived protein degradation was calculated as the ratio of TCA soluble medium to TCA-precipitated cell lysate radioactivity. Generation of AcGFP-NRBF2 HeLa-inducible cell line HeLa cells inducibly expressing AcGFP-NRBF2 was obtained using pTet-On Advanced system following the protocol manufacturer provided (Clontech Laboratories, Mount view, CA, USA). In brief, HeLa cells were firstly transfected with pTet-On Advanced Vector and selected withG418 to generate a stable Tet-On Advanced cell line. This cell line serves as the host for a TRE-Tight expression vector, which is transfected into the Tet-On Advanced cell line along with a linear Hygromycin marker. AcGFP-NRBF2 was inserted into MCS of TRE-Tight vector. After a second round of drug selection, a stable cell line is produced that expresses high level of the AcGFP-NRBF2 in response to doxycycline. Statistical analysis The values were expressed as mean±s.e.m. and P values <0.05 were considered significant. To analyse the differences between two groups, unpaired t -test was used if the distribution of value passed the normality test, otherwise Mann–Whitney U -test was used. For data normalized with control group (control is 1), one sample t -test against hypothetical value 1 was used to compare the difference between other group and control group. For multiple group comparison, if data pass the normal distribution test and homogeneity of variance test, multiple t -test followed by Bonferroni correction or one-way analysis of variance was used to analyse differences, otherwise Kruskal–Wallis test was used to analyse differences. All the tests are two-sided. All statistical analyses were performed using GraphPad Prism 5.0 or SPSS 20.0 software. How to cite this article: Lu, J. et al. NRBF2 regulates autophagy and prevents liver injury by modulating Atg14L-linked phosphatidylinositol-3 kinase III activity. Nat. Commun. 5:3920 doi: 10.1038/ncomms4920 (2014).